Laser printing of silicon nanoparticles with resonant optical electric and magnetic responses Silicon nanoparticles with sizes of a few hundred nanometres exhibit unique optical properties due to their strong electric and magnetic dipole responses in the visible range. Here we demonstrate a novel laser printing technique for the controlled fabrication and precise deposition of silicon nanoparticles. Using femtosecond laser pulses it is possible to vary the size of Si nanoparticles and their crystallographic phase. Si nanoparticles produced by femtosecond laser printing are initially in an amorphous phase (a-Si). They can be converted into the crystalline phase (c-Si) by irradiating them with a second femtosecond laser pulse. The resonance-scattering spectrum of c-Si nanoparticles, compared with that of a-Si nanoparticles, is blue shifted and its peak intensity is about three times higher. Resonant optical responses of dielectric nanoparticles are characterized by accumulation of electromagnetic energy in the excited modes, which can be used for the realization of nanoantennas, nanolasers and metamaterials. Control and manipulation of light on the micro- and nanoscales belong to the most challenging issues in modern optics. At sub-wavelength dimensions, metal nanostructures, nanoantennas and nanoparticles were investigated during recent years. They are characterized by strong resonant response to the electric field of light [1] , [2] , which appears due to excitation of collective electron oscillations known as localized surface plasmons. Interaction of the magnetic field component of light with matter is much weaker in nature [3] . Specially designed metallic nanostructures, such as pairs of nanorods or split-ring resonators, can however exhibit a magnetic dipole response, which is not found in naturally occuring materials. These nanostructures, usually forming the building blocks of metamaterials, are also called metaatoms [4] , [5] . Owing to their interaction with the magnetic field component of light, such artifical materials can have an effective permeability μ substantially deviating from unity, enabling the tunability of optical properties and realization of negative refractive indices [6] . However, at optical frequencies, metals have high non-radiative ohmic losses, leading to large absorption and unwanted heating effects, which limit applications of metal nanostructures in photonics. An alternative approach to control and manipulate light at nanoscale dimensions is based on high refractive index dielectric or semiconductor nanoparticles. It is well known from Mie theory that the first and second lowest resonances in the light-scattering spectrum of dielectric spheres in the frequency domain correspond to the magnetic and electric dipole terms [7] , [8] . The quality factors of these Mie resonances and their light-scattering efficiency stongly depend on the material refractive index. Owing to the resonant properties of high refractive index dielectric spherical particles, they were suggested as novel building blocks of dielectric metamaterials with negative effective permeability and permittivity [9] , [10] . The first experimental demonstrations of dielectric metamaterials with strong magnetic and electric responses in different spectral ranges from microwave to mid-infrared frequencies have been recently reported [9] , [11] . Fabrication of spherical dielectric nanoparticles and their arrangement in ordered metamaterial structures still remains a challenging problem. A suitable material with a high refractive index and small absorption coefficient, together with a novel fabrication technology are required. This technology should allow the generation of spherical nanoparticles with electric and magnetic Mie resonances in the visible spectral range as well as precise control over their sizes, shapes and positions. Nanoparticles of crystalline silicon (Si), the basic material of silicon photonics, provide a promising choice. Their optical properties and properties of Si nanoparticle arrays have been investigated theoretically [12] , [13] , [14] . Strong magnetic and electric resonant responses of spherical silicon nanoparticles in the visible and near-infrared spectral ranges have been experimentally demonstrated [15] , [16] . In these papers, Si nanoparticles were generated by femtosecond laser ablation from bulk Si targets without any control over the number of generated nanoparticles, their sizes and positions. Nanoparticle generation from bulk Si targets, including statistical properties of this process with respect to the number of generated nanoparticles and their size distribution, have been recently studied [17] . In this paper it was demonstrated for the first time that using a ring-shaped intensity distribution, single Si nanoparticles can be generated from bulk Si targets. Unfortunately, the minimum particle size that was obtained by this method was ~400 nm. These nanoparticles have dipole resonances in the infrared region of the spectrum. So far, there is no technology for the controlled generation of single spherical Si nanoparticles with the electric and magnetic dipole resonances in the visible spectral range. The above-mentioned problem is solved in this paper and a novel fabrication technique allowing the generation of individual spherical silicon nanoparticles with precisely controlled sizes, crystallographic phase and positions is demonstrated for the first time. This technology relies on femtosecond laser printing of Si nanoparticles onto a glass receiver substrate using silicon-on-insulator (SOI) wafers as laser targets and does not require any lithographic process. Nanoparticles generated by this method are initially in amorphous phase (a-Si). By additional single-pulse laser irradiation, the amorphous nanoparticles can be controllably transformed into crystalline particles (c-Si) or into particles with more complex mixed amorphous/crystalline phases, providing possibilities to tune optical properties of individual Si nanoparticles. These nanoparticles have electric and magnetic dipole Mie resonances in the visible spectral range, which can be used for the realization of efficient nanoantennas [18] , [19] , [20] , nanolasers and novel metamaterials. Fabrication technique Unique optical properties of silicon nanoparticles cannot be exploited and used without a simple method for their controlled fabrication. Chemical methods [10] , [21] , [22] , plasma synthesis [23] and laser ablation in air or liquids [17] , [24] , [25] can produce silicon nanoparticles with sizes in a broad range (from nm to μm), but without possibilities of the required size control and precise deposition of these nanoparticles. Lithographic methods [26] are more complex and do not allow the fabrication of spherical nanoparticles. In this paper, a new technique for the generation and positioning of silicon nanoparticles by femtosecond laser printing is developed. This method is based on laser-induced transfer of molten nanodroplets initiated by tightly focused laser pulses. A similar approach has already been applied to the controlled fabrication of metal nanoparticles [27] , [28] , [29] , [30] , [31] , [32] . A more sophisticated method using a ring-shaped femtosecond laser intensity distribution has been recently applied for the generation of single Si nanoparticles from bulk Si targets [17] . Unfortunately, in this case, the size of produced nanoparticles is larger than 400 nm. Much better control of the generated nanoparticles (in terms of their sizes and shape) can be obtained using SOI targets and tightly focused Gaussian laser pulses. In our experiments, SOI wafers with a single crystalline 50 nm silicon layer on 200 nm silicon oxide substrate are used for precise laser printing of Si nanoparticles (see Fig. 1a ). A commercial femtosecond laser system (Tsunami Femtosecond Oscillator and Spitfire Amplifier, Spectra Physics) is used, providing laser pulses at 800 nm central wavelength, with maximum pulse energies of up to 3 mJ, and pulse duration of 50 fs at the repetition rate of 1 kHz. For the controlled fabrication of Si nanoparticles, single laser pulses with an energy of about 5 nJ are used. Laser pulses are tightly focused by a long-distance microscope objective (Nikon) with × 50 magnification and a numerical aperture (NA) of 0.45. The long working distance of 17 mm allows irradiation of the target surface through the receiver glass substrate without noticeable distortion of the laser beam profile. According to the relation d = λ /(2NA), the estimated full-width at half-maximum diameter of the laser pulse focus is d =890 nm. 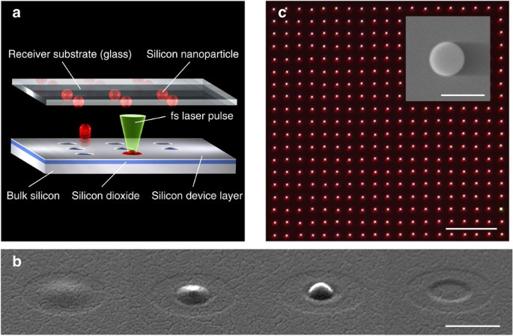Figure 1: Laser-printing process of Si nanoparticles. (a) Schematic illustration of femtosecond laser printing of nanoparticles. A silicon-on-insulator (SOI) wafer was used as a target to transfer spherical Si nanoparticles from 50 nm crystalline Si layer onto the transparent glass receiver substrate. (b) SEM images of the target before and after nanoparticle-ejection process from the SOI substrate. From left to right, the laser pulse energy is gradually increased. The last image shows the remaining hole in the silicon layer after the nanoparticle ejection (scale bar, 400 nm). (c) Array of several hundreds of amorphous Si nanoparticles (diameter of ≈160 nm) fabricated by this method and visualized with dark-field microscopy (scale bar, 20 μm). The insert shows a SEM image of a single Si nanoparticle in this array (scale bar, 200 nm). Figure 1: Laser-printing process of Si nanoparticles. ( a ) Schematic illustration of femtosecond laser printing of nanoparticles. A silicon-on-insulator (SOI) wafer was used as a target to transfer spherical Si nanoparticles from 50 nm crystalline Si layer onto the transparent glass receiver substrate. ( b ) SEM images of the target before and after nanoparticle-ejection process from the SOI substrate. From left to right, the laser pulse energy is gradually increased. The last image shows the remaining hole in the silicon layer after the nanoparticle ejection (scale bar, 400 nm). ( c ) Array of several hundreds of amorphous Si nanoparticles (diameter of ≈160 nm) fabricated by this method and visualized with dark-field microscopy (scale bar, 20 μm). The insert shows a SEM image of a single Si nanoparticle in this array (scale bar, 200 nm). Full size image During illumination of the SOI wafer by a single tightly focused Gaussian laser pulse, absorption in the top Si layer leads to ultrafast heating and local melting of this layer. The oxide substrate (melting temperature of which is much higher) remains unaffected at these laser pulse energies. The liquid phase of silicon has higher density compared with its solid phase, leading to a volume reduction induced by melting. Depending on the laser pulse energy on the SOI surface, different scenarios can be observed, as demonstrated in a sequence of scanning electron microscope (SEM) images shown in Fig. 1b . At low pulse energies, the silicon layer is not completely melted through its thickness ( Fig. 1b left). Owing to the surface tension, the molten region contracts to the centre and forms a semispherical bump (two middle images in Fig. 1b ). At higher laser pulse energies, the 50 nm silicon layer melts completely forming a droplet induced by the surface tension. This droplet formation is accompanied by the elevation of its centre-of-mass. The generated spherical droplet acquires an upward-directed momentum, which drives it towards the receiver substrate placed on top of the SOI wafer, where the liquid material solidifies at the surface. The described process is performed in air at atmospheric pressure and the distance between the receiver and the donor substrate is set to ~5 μm. Right image in Fig. 1b shows the remaining cavity in the silicon layer after the droplet ejection. From this image, the diameter of the molten area can be estimated to be ~250 nm. Taking into account the 50 nm Si layer thickness, the liquid disk volume transforms into a spherical droplet with a diameter of ~160 nm. Thus, the Si layer thickness is one of the parameters allowing controlling the size of generated nanoparticles. An example of a printed large array of Si nanoparticles with 160 nm diameter and periodicity of 5 μm is shown in Fig. 1c as a dark-field microscopic image. The insert provides a SEM image of a single Si nanoparticle in this array, obtained in a low-vacuum mode to avoid conductive coating, which is usually required for SEM imaging. One can vary the nanoparticle diameter by increasing the laser pulse energy in steps of ~0.1 nJ starting from 5 nJ. SEM images of the obtained nanoparticles are shown in Fig. 2a . The diameters of these particles can be adjusted in the range of 160–240 nm and their dark-field microscopic images are given in Fig. 2b . 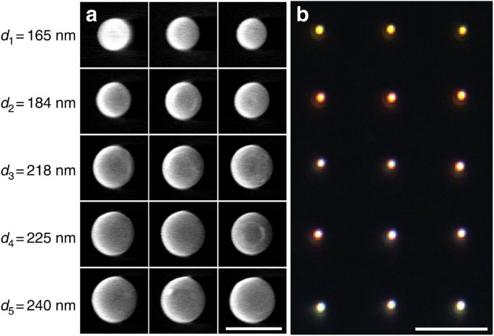Figure 2: Laser pulse energy dependence of the nanoparticle diameter. (a) SEM images of nanoparticles fabricated at slightly different laser pulse energies starting from 5 nJ. Each line, from top to bottom, corresponds to the laser pulse energy increase of ~0.1 nJ (scale bar, 300 nm). (b) Changes in the optical response of the generated nanoparticles are visualized by dark-field microscopic images (scale bar, 5 μm). The given nanoparticle diameters represent an average value with a deviation of ±5 nm. Figure 2: Laser pulse energy dependence of the nanoparticle diameter. ( a ) SEM images of nanoparticles fabricated at slightly different laser pulse energies starting from 5 nJ. Each line, from top to bottom, corresponds to the laser pulse energy increase of ~0.1 nJ (scale bar, 300 nm). ( b ) Changes in the optical response of the generated nanoparticles are visualized by dark-field microscopic images (scale bar, 5 μm). The given nanoparticle diameters represent an average value with a deviation of ±5 nm. Full size image Optical characterization Optical characterization of the fabricated single Si nanoparticles has been performed by an optical fiber spectrometer (HR 2000, Ocean Optics), which was connected to a dark-field microscope setup. A dark-field condenser (Mueller Optronic, NA=0.9) was used to illuminate Si nanoparticles from bottom through the glass substrate. The light scattered by individual nanoparticles is imaged by a microscope objective with × 50 magnification and a NA of 0.55 (Zeiss) simultaneously on a CCD (charge-coupled device) camera and an optical fibre facette with an aperture of 200 μm. This setup allows to collect the light scattered by a single particle. The scattering spectrum of a single Si nanoparticle deposited on a glass substrate directly after laser printing is shown in Fig. 3a (blue curve). The spectrum exhibits two resonance peaks. A comparison with the scattering spectrum calculated using Mie theory (red curve) for a spherical Si nanoparticle with diameter of 161 nm (taken from the experimental results) reveals that the laser-printed particle is in amorphous phase and that the observed resonances correspond to magnetic ( λ ≈720 nm) and electric ( λ ≈590 nm) dipole scattering. The glass substrate does not affect the spectral positions of the optical resonances for spherical Si nanoparticles compared with a homogeneous environment [15] . The spectral positions are determined by the dielectric permittivity of the particle material and the particle size. If the shape of the printed nanoparticles significantly differs from a sphere, spectral positions of the magnetic and electric dipole resonances will not correspond to the presented Mie simulations. This fact confirms the conclusion about the spherical shape of the printed nanoparticles. For crystalline Si nanoparticles with the same sizes, positions of resonances are blue shifted and the scattering efficiency is increased, as can be seen in Fig. 3b,c (red curves). In calculations of scattering spectra of nanoparticles with mixed crystallographic phases, their dielectric functions are taken as a sum of crystalline and amorphous Si dielectric functions multiplied by a fitting parameter corresponding to the fractions of these phases in the nanoparticle volume. 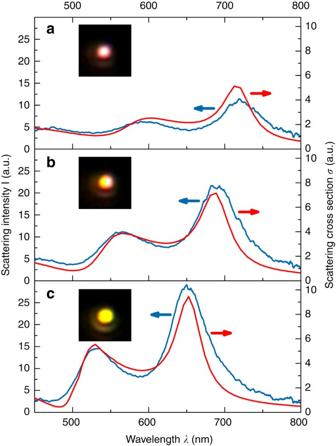Figure 3: Scattering properties of Si nanoparticles with different crystallographic phases. Experimental (blue curves) and theoretical (red curves) scattering spectra, calculated using Mie theory, of spherical Si nanoparticles. The inserts demonstrate dark-field microscopic images of the corresponding Si nanoparticles. (a) Experimental scattering spectrum of laser-printed Si nanoparticle. The theoretical spectrum is calculated for an amorphous Si nanoparticle with diameter of 161 nm. (b) The printed Si nanoparticle is irradiated by a second laser pulse with low energy. The theoretical spectrum is calculated for a 70% crystalline Si nanoparticle with diameter of 166 nm. (c) The printed Si nanoparticle is irradiated by a second laser pulse with high pulse energy. The theoretical spectrum is calculated for a pure crystalline Si nanoparticle with diameter of 163 nm. The dielectric functions for amorphous and crystalline silicon are taken from ref.44. Figure 3: Scattering properties of Si nanoparticles with different crystallographic phases. Experimental (blue curves) and theoretical (red curves) scattering spectra, calculated using Mie theory, of spherical Si nanoparticles. The inserts demonstrate dark-field microscopic images of the corresponding Si nanoparticles. ( a ) Experimental scattering spectrum of laser-printed Si nanoparticle. The theoretical spectrum is calculated for an amorphous Si nanoparticle with diameter of 161 nm. ( b ) The printed Si nanoparticle is irradiated by a second laser pulse with low energy. The theoretical spectrum is calculated for a 70% crystalline Si nanoparticle with diameter of 166 nm. ( c ) The printed Si nanoparticle is irradiated by a second laser pulse with high pulse energy. The theoretical spectrum is calculated for a pure crystalline Si nanoparticle with diameter of 163 nm. The dielectric functions for amorphous and crystalline silicon are taken from ref. 44 . Full size image Laser-induced crystallization Laser-induced crystallization of amorphous semiconductors is an important topic in material science [33] , [34] , [35] . To induce a crystallographic phase transition in amorphous nanoparticles, additional single-pulse laser irradiation of these particles is applied. For this purpose the same femtosecond laser system is used. To achieve homogeneous and reproducible crystallization of nanoparticles, they are irradiated by a single femtosecond laser pulse with a flat-top intensity distribution and a laser pulse energy of 58 nJ. This distribution is realized by imaging of a square-shaped aperture (250 μm × 250 μm) onto the sample surface. After a × 50 demagnification, the size of the obtained square-shaped intensity distribution is 5 μm × 5 μm. Crystallization of laser-printed Si nanoparticles is immediately visible in their scattering spectra ( Fig. 3b,c ). The direct proof of crystallinity of a Si nanoparticle, similar to that investigated in Fig. 3c , is provided in Fig. 4 showing a transmission electron microscope image of this nanoparticle. One can clearly see parallel lines corresponding to the atomic lattice proving monocrystallinity of this particle. 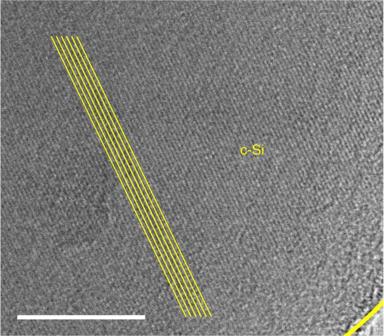Figure 4: TEM image of a monocrystalline Si nanoparticle. Yellow lines are added for better visibility of the atomic lattice. The nanoparticle surface can be seen in the lower right corner indicated by a yellow line (scale bar, 10 nm). Figure 4: TEM image of a monocrystalline Si nanoparticle. Yellow lines are added for better visibility of the atomic lattice. The nanoparticle surface can be seen in the lower right corner indicated by a yellow line (scale bar, 10 nm). Full size image Scattering signal produced by crystallized nanoparticles is much stronger and they appear in different colour compared with non-irradiated amorphous particles as can be seen in Fig. 3 (see inserts). This process provides possibilities for the generation of silicon nanoparticles with adjustable optical properties (see Fig. 3b,c ). Moreover, application of laser-induced crystallization in an array of amorphous Si nanoparticles allows selective crystallization of single nanoparticles. Results of such selective crystallization are shown in Fig. 5 . 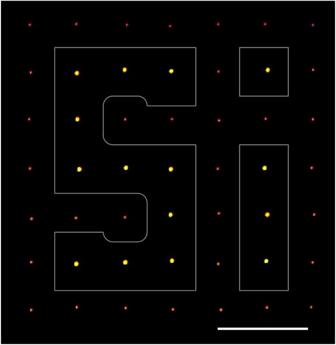Figure 5: Dark-field microscopic image of the laser-printed Si nanoparticles. The nanoparticles within the white lines are crystallized by additional laser pulse irradiation, producing a visible colour change (scale bar, 10 μm). Figure 5: Dark-field microscopic image of the laser-printed Si nanoparticles. The nanoparticles within the white lines are crystallized by additional laser pulse irradiation, producing a visible colour change (scale bar, 10 μm). Full size image In this section the origin of the magnetic dipole resonance is discussed. It is proved by a simple theoretical consideration that the magnetic dipole resonance of Si nanoparticles is indeed excited by the magnetic field component of light due to Faraday’s law of electromagnetic induction. One can find different statements concerning this subject [16] , [36] . We consider a spherical particle with the dielectric constant ε p located in a homogeneous magnetic field H 0 ( t )= H 0 exp(− iωt ) oscillating in time with the frequency ω . One can use the so-called quasi-static approximation [3] , [37] to calculate magnetic field outside the particle. Inside the particle, the polarization current j = ∂ D / ∂t =− iωε 0 ε p E , where D = ε 0 ε p E is the electric induction and ε 0 is the vacuum dielectric constant. E is the electric field inside the particle induced by the time-varying total magnetic field due to Faraday’s law ∇ × E = iωμ 0 H , where μ 0 is the vacuum permeability. The case of a metallic particle located in time-oscillating magnetic field has been considered in ref. 3 . It has been shown that the magnetic field scattered by the metallic particle is equivalent to that produced by a magnetic dipole m = α m H 0 with the polarizability where V is the particle volume and r is its radius, k is the wavenumber inside the particle ( k 2 = ω 2 μ 0 ε 0 ε p ). This expression coincides with the magnetic dipole polarizability, which can be obtained from Mie theory in the limit r / λ <<1 (refs 11 , 38 , 39 , 40 ). If equation (7) is applied to dielectric particles with a negligibly small imaginary part of ε p , resonances at rk = πl , where l is an integer number, appear. At these resonances, the magnetic polarizability, induced by the external magnetic field, diverges. The reason is that in the quasi-static approximation, all propagating radiation terms are omitted. Taking them into account, we get the following expression for the magnetic polarizability of a small nanoparticle ( r / λ <<1) where k 0 is the wavenumber in free space . The derivation of this expression is presented in the Methods section. Both expressions for the magnetic polarizability coincide in case of k 0 →0. Note that for dielectric nanoparticles, radiation loss is the main physical mechanism providing energy conservation in the light-scattering process, which always has to be taken into account. In Fig. 6 , the magnetic polarizabilities of a spherical Si nanoparticle with a radius of 65 nm calculated using the above expressions and Mie theory are compared. Without taking into account radiation losses equation (7), coincidence with Mie theory is poor, the resonance is narrow and its position is shifted to the blue side ( Fig. 6a ). Much better agreement is obtained between equation (2) and Mie theory ( Fig. 6b ). Moreover, at the resonant condition, the magnitudes and distributions of electric and magnetic fields inside the Si nanoparticle calculated using the above approach, that is, as a reaction on the magnetic field, and Mie theory coincide ( Fig. 7 ). These results demonstrate that the magnetic dipole resonance appears due to interaction between the dielectric nanoparticle and the magnetic field component of incident radiation. Note that the resonant optical responses of dielectric nanoparticles are accompanied by an accumulation of electromagnetic energy in the excited modes [15] , which can be used for the realization of effective nanoantennas and nanolasers. 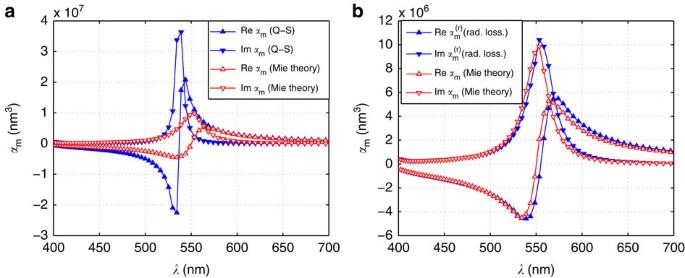Figure 6: Magnetic dipole polarizability of spherical Si nanoparticles. (a) Magnetic dipole polarizabilityαmcalculated using the quasi-static (Q–S) approach equation (7) and Mie theory. (b) Magnetic dipole polarizabilityαmcalculated using Mie theory and equation (2) taking into account radiation losses (rad. loss.). Dielectric permittivity for crystalline silicon is used44. The nanoparticle radius is equal to 65 nm. Figure 6: Magnetic dipole polarizability of spherical Si nanoparticles. ( a ) Magnetic dipole polarizability α m calculated using the quasi-static (Q–S) approach equation (7) and Mie theory. ( b ) Magnetic dipole polarizability α m calculated using Mie theory and equation (2) taking into account radiation losses (rad. loss.). Dielectric permittivity for crystalline silicon is used [44] . The nanoparticle radius is equal to 65 nm. 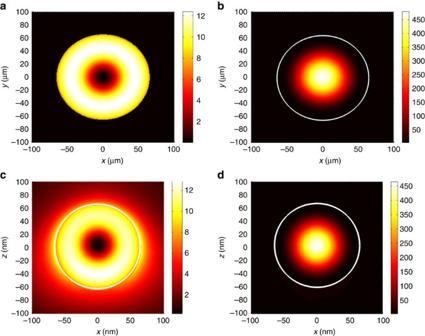Figure 7: Distributions of electric and magnetic fields inside a Si nanoparticle. Electric (a) and magnetic (b) field intensities calculated inside the nanoparticle as a reaction on magnetic field. Electric (c) and magnetic (d) field intensities calculated using Mie theory. The field intensities are presented in the cross-section of the nanoparticle with the radius of 65 nm. They are calculated in the plane perpendicular to the external magnetic field at the condition of magnetic dipole resonance. The white circles indicate the boundary of the nanoparticle. Full size image Figure 7: Distributions of electric and magnetic fields inside a Si nanoparticle. Electric ( a ) and magnetic ( b ) field intensities calculated inside the nanoparticle as a reaction on magnetic field. Electric ( c ) and magnetic ( d ) field intensities calculated using Mie theory. The field intensities are presented in the cross-section of the nanoparticle with the radius of 65 nm. They are calculated in the plane perpendicular to the external magnetic field at the condition of magnetic dipole resonance. The white circles indicate the boundary of the nanoparticle. Full size image Scattering diagrams of the resonant silicon nanoparticles are determined by interference of electromagnetic waves generated by the electric and magnetic dipoles. It has been shown theoretically that the backscattering of resonant silicon nanoparticles with a radius of 65 nm is totally suppressed at the light wavelength λ =590 nm [12] , also known as Kerker’s type zero backscattering [41] . This effect is realized when ε 0 α m = α p , where α m and α p are the magnetic and electric dipole polarizabilities of the nanoparticle. Directional light scattering by spherical silicon nanoparticles in the visible spectral range has been recently experimentally demonstrated [42] , [43] . This effect can be used for efficient light coupling into silicon waveguides. In conclusion, femtosecond laser printing of silicon nanoparticles onto a glass receiver substrate using SOI wafers as laser targets has been developed. The laser-printed nanoparticles can be arranged in periodic and more complex structures. The demonstrated novel fabrication technology allows the generation of individual amorphous and crystalline spherical Si nanoparticles with precisely controlled optical properties. The laser-printed nanoparticles are initially in amorphous phase (a-Si). By additional single-pulse laser irradiation, the amorphous nanoparticles can be controllably transformed into crystalline particles (c-Si) or into particles with more complex mixed amorphous/crystalline phases. This technology provides unique possibilities for laser tuning of optical properties of individual Si nanoparticles. These nanoparticles have electric and magnetic dipole Mie resonances in the visible spectral range, which can be used for the realization of efficient nanoantennas, nanolasers and novel metamaterials. The fact that the size and the crystallographic phase can be controllably influenced enables the fabrication of optical elements with laterally varying optical properties. We believe that the presented laser-printing technology and generated Si nanoparticles will find many applications in silicon photonics. Theoretical derivations The mechanism of the resonant interaction between Si nanoparticles with magnetic field of light can be clarified by considering the following electromagnetic problem: a particle with the dielectric constant ε p is located in a spatially uniform, time-oscillating magnetic field H 0 ( t )= H a exp(− iωt ). This case corresponds to the quasi-static approximation [3] , [37] , where the particle is much smaller than the electromagnetic wavelength λ . Here H a is the magnetic field amplitude and ω is the circular frequency. In the quasi-static approximation, the contribution of the displacement current to Ampere’s law [37] in the vicinity of nanoparticle can be neglected. Thus, the total magnetic field H ( e ) outside the particle satisfies the following equations Inside the particle, the displacement current j = ∂ D / ∂t =− iωε 0 ε p E ( D = ε 0 ε p E is the displacement vector, ε 0 is the vacuum dielectric constant, E is the electric field inside the particle induced by time-varying magnetic field due to Faraday’s law ∇ × E = iωμ 0 H , μ 0 is the vacuum permeability) cannot be neglected because its value depends on ε p . With the increasing ε p , the effective electromagnetic wavelength in the particle decreases making the retardation effects important. Thus, inside the particle the equations for the magnetic field are given by where k 2 = ω 2 μ 0 ε 0 ε p . Only if L 2 | ε p |/ λ 2 <<1 is satisfied, where L is the largest particle size, one can neglect the displacement current inside the particle. Using equations(3) and (4) and applying the field boundary conditions on the particle surface, one can find the total magnetic field in the system. Analytical solution of this problem is given in ref. 3 . The magnetic field H ( i ) ( r ) inside the particle can be written in the following form [3] where β is the unknown constant, which has to be found from the boundary conditions, r is the radius vector, n is the unit vector directed along r − r p ( r p is the radius vector of the particle centre), nn is the dyadic product, R =| r − r p |, Û is the unit 3 × 3 tensor, A ( R )=([ kR cos kR −sin kR ]/ R 3 +[ k 2 sin kR ]/ R ) and B ( R )=(3[ kR cos kR −sin kR ]/ r 3 +[ k 2 sin kR ]/ R ). The total magnetic field H ( e ) outside the particle is presented as a superposition of the external field H 0 and the field H p generated by the particle where α m H 0 = m is the magnetic dipole moment of the particle with its magnetic dipole polarizabilty α m , is the near-field (quasi-static) Green tensor. On the particle surface, all components of the total magnetic field have to be continuous. From this boundary condition we obtain where V =4 πa 3 /3 is the particle volume and a is its radius. For dielectric particles with negligibly small imaginary part of ε p , ak has only real values. Formally, the resonant condition in equation (7) is determined by ak = πl , where l =1, 2, 3, ….. The polarizability (7) coincides with the magnetic dipole polarizability obtained from Mie theory in the approximation a / λ <<1 (ref. 38) [38] . For dielectric particles, the polarizabity (7) diverges at the resonant conditions because the model does not take into account radiative damping. Note that radiative losses have to be always taken into account to fulfil energy conservation in the system with dielectric particles. In this case, the magnetic field H p around the particle should include not only the near-field part, as in equation (6), but also all retardation terms [12] . In framework of this approach, the magnetic field generated by the particles can be written as , where k 0 is the wavenumber in the surrounding medium, is the total Green tensor of the system without particles [12] . In the near-field region around the particle with ak 0 <<1, keeping the first two terms dependent on k 0 , we obtain Replacing the near-field tensor in (6) by the tensor (9) and applying the boundary conditions, the magnetic dipole polarizabilty can be written as How to cite this article: Zywietz, U. et al . Laser printing of silicon nanoparticles with resonant optical electric and magnetic responses. Nat. Commun. 5:3402 doi: 10.1038/ncomms4402 (2014).